Fractal free energy landscapes in structural glasses Glasses are amorphous solids whose constituent particles are caged by their neighbours and thus cannot flow. This sluggishness is often ascribed to the free energy landscape containing multiple minima (basins) separated by high barriers. Here we show, using theory and numerical simulation, that the landscape is much rougher than is classically assumed. Deep in the glass, it undergoes a ‘roughness transition’ to fractal basins, which brings about isostaticity and marginal stability on approaching jamming. Critical exponents for the basin width, the weak force distribution and the spatial spread of quasi-contacts near jamming can be analytically determined. Their value is found to be compatible with numerical observations. This advance incorporates the jamming transition of granular materials into the framework of glass theory. Because temperature and pressure control what features of the landscape are experienced, glass mechanics and transport are expected to reflect the features of the topology we discuss here. Understanding the dynamics of glasses is one of the oldest and most challenging problems in the theory of matter. The classical thermodynamic picture interprets the slow relaxation of glasses in terms of a free energy landscape with fairly simple structural features ( Fig. 1 ): each minimum is a stable amorphous glass state, high frequency relaxations correspond to vibrational excitations of the state and slow relaxations correspond to jumps between different states [1] , [2] , [3] . Yet experimental and numerical observations suggest that this simple landscape description—with essentially only one type of barrier—is insufficient to capture the complexity of glassy dynamics. Low-temperature glasses exhibit an intermediate slow (Johari-Goldstein) relaxation whose timescale is indeed difficult to interpret as one corresponding to jumps between widely different states [4] . It has thus been proposed that the landscape features narrow sub-basins, separated by small barriers, that aggregate into wider metabasins, separated by large barriers ( Fig. 1 ). Johari-Goldstein relaxation processes would then connect sub-basins within a same metabasin [4] , [5] . Direct numerical investigations have confirmed the metabasin organization and thereby improved the phenomenological description of transport [6] , [7] . Deep within the glass phase, the out-of-equilibrium dynamics is also unable to properly sample the distribution of barriers associated with the complex sub-basin structure, which could explain why describing it with a single fictive temperature is not possible [8] , [9] . 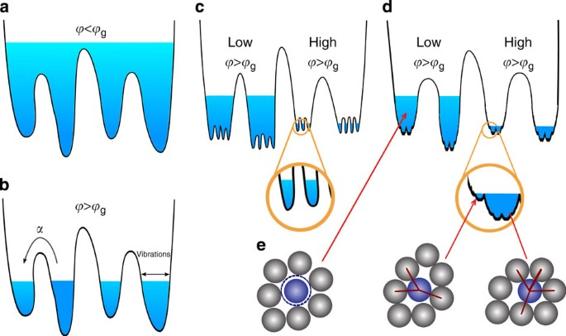Figure 1: Free energy landscape with simple basins, metabasins and fractal basins. Schematic depictions of (a) the liquid state at packing fractionsϕthat are smaller than the glass transitionϕg, and of free energy basins for different landscape scenarios: (b) simple stable basins, (c) metabasins of sub-basins (d) and metabasins of marginal basins. The simple landscape description is akin to boating on a system of lakes separated by high mountains. In the liquid, all of space can be explored. At lower water levels, each basin is a different glass. The free energy barriers hinder passing from one glass to another (the so-calledα-relaxation); the basin width allows for vibrational relaxation. Both incandd, the water level further determines what features of the landscape are experienced. Deep into the glass, the landscape roughness results in intra-state barriers that are associated with secondary relaxations. Ind, at very low water levels (right)—deep into the fractal glass—lakes transform into a complex wetland with a hierarchy of small ponds. (e) The very bottom of each of these ponds corresponds to a given realization of the force network (red lines), but the identification of the force contacts remains undetermined before the fractal regime is reached (dashed line). Figure 1: Free energy landscape with simple basins, metabasins and fractal basins. Schematic depictions of ( a ) the liquid state at packing fractions ϕ that are smaller than the glass transition ϕ g , and of free energy basins for different landscape scenarios: ( b ) simple stable basins, ( c ) metabasins of sub-basins ( d ) and metabasins of marginal basins. The simple landscape description is akin to boating on a system of lakes separated by high mountains. In the liquid, all of space can be explored. At lower water levels, each basin is a different glass. The free energy barriers hinder passing from one glass to another (the so-called α -relaxation); the basin width allows for vibrational relaxation. Both in c and d , the water level further determines what features of the landscape are experienced. Deep into the glass, the landscape roughness results in intra-state barriers that are associated with secondary relaxations. In d , at very low water levels (right)—deep into the fractal glass—lakes transform into a complex wetland with a hierarchy of small ponds. ( e ) The very bottom of each of these ponds corresponds to a given realization of the force network (red lines), but the identification of the force contacts remains undetermined before the fractal regime is reached (dashed line). Full size image A disordered ensemble of (nearly) hard spheres, that is, spherical particles that cannot overlap, is often taken as a simple model for glasses, both in theoretical and experimental studies. The behaviour of static assemblies of macroscopic spheres [10] , colloidal suspensions [11] , [12] , [13] and dynamically agitated ensembles of grains [14] is indeed akin to that of thermal glasses. Like thermal glasses, hard spheres can also be theoretically described in terms of a complex free energy landscape dominated by entropic effects [15] ; the same analysis tools can be used for both systems [16] , underlying the similarity of their dynamical behaviour [17] and of their phase diagram in terms of pressure and density [18] . In addition, when hard sphere interactions are considered, a new kind of geometric phase transition appears, the jamming transition [19] , [20] , [21] , that can be characterized in two equivalent ways. From a thermodynamic point of view, compressing a hard sphere glass to infinite pressure results in an amorphous jammed packing in which particles are completely arrested and mechanically equilibrated [18] . From a rheological point of view, hard sphere glass rigidity is entropic before reaching the jamming transition, and (relaxing the harshness of the hard sphere repulsion) mechanical beyond jamming, as in low-temperature molecular glasses [22] . On approaching jamming, hard sphere glasses are marginally stable [23] , [24] , [25] : they have very soft vibrational modes and excitations that extend over a wide range of timescales [19] , [25] and can be characterized in terms of critical scalings similar to ordinary phase transitions, see refs 20 , 21 for reviews. The critical properties of the jamming transition hence provide additional insights into the structure of the landscape. Yet neither the marginality of the basins nor the smallness of the barriers associated with the soft modes fit in the simple landscape picture [18] , which is hence unable to explain the critical properties of the jamming transition. In the late eighties, Kirkpatrick, Thirumalai and Wolynes proposed that mean-field disordered models contain the essential features of glassy landscapes [26] , [27] , [28] . These models fall in two broad universality classes: the so-called Random First Order (the simple picture of a stable glass, with featureless basins and large barriers) [26] , [27] and another class where one large state is broken up in a fractal hierarchy of basins within basins, discovered by one of us in the Sherrington-Kirkpatrick (SK) model [29] , [30] . The first class yields, close to the glass transition, a two-step dynamical relaxation [31] in the same universality class as the mode-coupling theory [17] , [32] . It was thus taken to represent (fragile) structural glasses, at least close to the glass transition—hence the name Random First Order Transition (RFOT) associated with this proposal. Gardner, however, introduced a twist to this classification [33] . She found that, when continued deep in the glass phase, RFOT systems generically reach another phase transition. At this transition, each individual amorphous state (basin) becomes a metabasin by breaking into a full fractal hierarchy of sub-basins akin to that of the SK model, while retaining its identity as a metabasin. Surprisingly, despite an early comment to the effect that this ‘fractal phase’ might be related to secondary relaxations in real glasses [26] , it has since remained somewhat of an intellectual curiosity. Although the RFOT scenario was initially proposed as an analogy, today we know it to be exact for particles in the limit of large spatial dimensions d (refs 34 , 35 , 36 ). Solving a problem through an expansion around the limit d →∞ is an established strategy in quantum mechanics, atomic physics and statistical mechanics when there are no small parameters [37] , [38] , and the glass problem is no exception. The question whether a given feature is captured by RFOT then becomes whether that same feature extrapolates continuously from d =3 to d →∞, a fact that may be checked with numerical simulations. It is numerically found that the main features of the bottom of the basins, which are related to jamming, are extremely stable with varying dimension [39] , [40] , [41] ; note by contrast that the behaviour of high barriers, which are connected to the relaxation around the glass transition, remains the object of lively debates [2] , [42] , [43] . The main object of this paper is to report that the exact hard sphere solution in the limit d →∞ predicts the existence of a Gardner transition to a fractal phase in the glass regime, and that taking this transition into account is crucial to understanding the physics of jamming ( Fig. 1 ). It affects the out-of-equilibrium dynamics deep in the glass phase [9] , [44] , [45] , [46] , incorporating (at least partially) secondary relaxations, a point that we here only briefly touch upon. Sub-basins and barriers of a wide variety of sizes also bring along marginality and soft modes, features that were absent in the original RFOT scenario. Their inclusion allows us to make contact with and incorporate the features of jamming theory associated with marginality and isostaticity [23] , [24] , [25] . More specifically, we show that (i) the marginal and fractal phase deep inside hard sphere glasses fully contains the jamming transition; (ii) taking this result into account, one can make analytic predictions for the critical exponents of the jamming transition that are fully compatible with observations; and (iii) one can compute the probability distribution of the forces in jammed packings, which displays an analogue of the Coulomb gap [47] , resulting in a power-law scaling of the distribution of small forces [40] , [48] . Because the critical properties of jamming are independent of spatial dimension [39] , [40] , [41] , the results obtained in d →∞ immediately translate to experimental systems in d =2, 3 and hence provide a first unambiguous application of the fractal phase in finite dimension. Phase diagram Using an approach similar to that used for solving the SK model, the exact d →∞ solution for d -dimensional identical hard spheres of unit diameter can be formulated in terms of a caging order parameter Δ( y ) (refs 29 , 30 ). This functional order parameter, which encodes the width Δ of metabasins on a (properly defined) scale y , is obtained by numerically solving a set of integro-differential equations ( Supplementary Note 1 ) and then used to calculate the theoretical liquid–glass phase diagram ( Fig. 2 ). The theory predicts that a compressed liquid falls out of equilibrium and becomes a glass at a pressure that depends on the compression rate. Once in a glass state, further compression results in a quick increase of the system pressure p , and on jamming p →∞ (ref. 18 ). The final jamming density depends on compression speed, hence defining a J-line of jammed states [18] . Two examples of glass compression obtained using an approximate state following are reported in Fig. 2 (ref. 49 ). 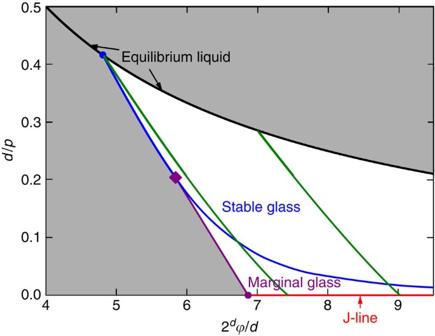Figure 2: Phase diagram of infinite-dimensional amorphous hard spheres. Pressurep—packing fractionϕphase diagram ford→∞ hard spheres. The white region indicates the regime where the (meta)basin structure is present, either as a simple stable glass or as a marginal fractal glass. The left-most boundary of the glass region is the threshold line. The ‘J-line’ of jammed packings is found alongp=∞, which always falls within the marginal phase. Although solving the mean-field out-of-equilibrium dynamics of hard spheres remains an open problem, an adiabatically slow compression should leave the equilibrium liquid line and eventually reach the J-line, while remaining within the white region. The green lines are two examples of an adiabatic following of a glass state18. Figure 2: Phase diagram of infinite-dimensional amorphous hard spheres. Pressure p —packing fraction ϕ phase diagram for d →∞ hard spheres. The white region indicates the regime where the (meta)basin structure is present, either as a simple stable glass or as a marginal fractal glass. The left-most boundary of the glass region is the threshold line. The ‘J-line’ of jammed packings is found along p =∞, which always falls within the marginal phase. Although solving the mean-field out-of-equilibrium dynamics of hard spheres remains an open problem, an adiabatically slow compression should leave the equilibrium liquid line and eventually reach the J-line, while remaining within the white region. The green lines are two examples of an adiabatic following of a glass state [18] . Full size image Independently of compression rate, the glass basin in which the system is initially trapped undergoes a Gardner transition [33] , at a line computed in ref. 36 . Our key result is that, at pressures above this line, basins transform into metabasins that contain a collection of marginally stable glasses, a phenomenon that is described by a non-trivial caging order parameter Δ( y ) as in the SK model [29] . Finding the solution that describes the marginal phase allows us to delimit the marginal phase boundary ( Supplementary Note 1 ) to within the Gardner transition line of ref. 36 , the J-line and the ‘threshold’ line determined following the prescription of ref. 46 . The fact that within this region at least one eigenvalue of the stability matrix in the free energy space vanishes confirms that this phase is indeed marginally stable ( Supplementary Note 1 ) [50] . We also find that, while the radius of the innermost fractal basins shrinks to zero as a power-law Δ EA ~ p −κ (see below), the radius of the largest metabasins remains of order one. Close to jamming, the total entropy of a group of metabasins of width Δ grows as Δ 1/κ , hence the basins have a phase space structure whose fractal dimension is 2/κ (see Supplementary Note 1 for a more detailed discussion). The marginal phase is thus also fractal. The existence of the marginal phase can be qualitatively tested by molecular dynamic (MD) numerical simulations in finite d ( Supplementary Note 2 ) by considering the outcome of a slow compression from the liquid up to jamming [40] , [51] . Jammed systems are isostatic, and thus particles have an average of 2 d force-bearing neighbours [19] , [25] , [40] , [52] , [53] , [54] , which is much smaller than the ( e d ) neighbours that isotropically cage a particle in an equilibrated dense liquid. Because the identity of the force-bearing neighbours at jamming uniquely characterizes the state, their emergence sensitively depends on the landscape structure ( Fig. 1 ). In the simple basin scenario, force-bearing neighbours at jamming should be fully determined immediately on leaving the equilibrium liquid; in the meta/sub-basin scenario, that determination should only occur once sufficiently deep in the glass for transitions between sub-basins to be fully suppressed; in a fractal phase, by contrast, the contacts should be gradually determined as jamming is approached. To test this scenario, we consider a glass configuration at pressure p init . Starting from this configuration, we perform several independent compressions up to p f =10 10 and for each compressed configuration we measure the force network. We obtain a set of contact variables , which are set to unity if particles i and j form a force-bearing contact in configuration a and to zero otherwise. The average of over pairs ab of compressed configurations and over contacts ij provides a measure of similarity between the force networks. The fact that this quantity increases smoothly on increasing p init indicates that the force network is only partially encoded in the initial configuration, in support of the fractal landscape scenario ( Fig. 3a and Supplementary Note 2 ). 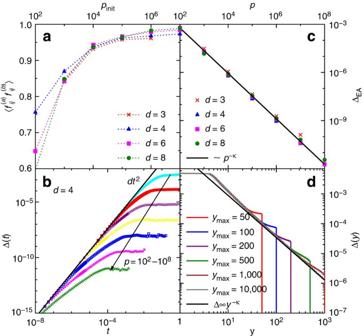Figure 3: Force network and position overlaps in the fractal basin. (a) Overlap between the force network edgesfij=0, 1 that connect two particlesiandjin two glass configurationsaandb(at pressurepf=1010), obtained by independent compression of the same initial configuration at initial pressurepinit(Supplementary Note 2). (b) Time-evolution of the mean-square displacement Δ(t) for glasses atp=102, 103, 104, 105, 106, 107and 108ind=4. The solid line indicates the ballisticdt2behaviour. The long-time value is the cage sizedΔEA. (c) The pressure evolution of the cage size ΔEAin various dimension closely follows a power-law ~p−κwith the theoretical value κ =1.41575. (d) Analytical results for the order parameter Δ(y) at 2d. Increasing the cutoffymax~pindicates that the scaling regime Δ(y)~y−κextends to ally. (Supplementary Note 1) Figure 3: Force network and position overlaps in the fractal basin. ( a ) Overlap between the force network edges f ij =0, 1 that connect two particles i and j in two glass configurations a and b (at pressure p f =10 10 ), obtained by independent compression of the same initial configuration at initial pressure p init ( Supplementary Note 2 ). ( b ) Time-evolution of the mean-square displacement Δ( t ) for glasses at p =10 2 , 10 3 , 10 4 , 10 5 , 10 6 , 10 7 and 10 8 in d =4. The solid line indicates the ballistic dt 2 behaviour. The long-time value is the cage size d Δ EA . ( c ) The pressure evolution of the cage size Δ EA in various dimension closely follows a power-law ~ p −κ with the theoretical value κ =1.41575. ( d ) Analytical results for the order parameter Δ( y ) at 2 d . Increasing the cutoff y max ~ p indicates that the scaling regime Δ( y )~ y −κ extends to all y . ( Supplementary Note 1 ) Full size image Criticality of the jamming transition The equations that describe the marginal phase are formulated in terms of the caging order parameter Δ( y ) and the pair correlation function g ( r ), which also encodes the probability distribution of forces in the packing. On approaching the J-line, that is, as a hard sphere glass approaches p →∞, these equations develop a scaling regime ( Fig. 3d ) that is characterized by three main critical exponents: θ for the weak forces, α for the quasi-contacts and κ for Δ itself. A (non-trivial) generalization of the approach developed for the SK model [55] allows us to obtain theoretical values for these exponents ( Supplementary Note 1 ). Interestingly, the condition that fixes their value is precisely equivalent to the marginal stability condition. The theory therefore predicts that the criticality of the jamming transition directly follows from its location inside the marginal phase. A striking signature of marginality is the scaling of the innermost basin width captured by the Edwards-Anderson cage size Δ EA ~ p −κ . Although κ=3/2 was proposed in earlier studies [23] , [25] , [56] , the theory predicts a slightly smaller κ=1.41574 that is in remarkable agreement with our numerical results ( Fig. 3c ). Because single-particle caging by immediate neighbours (a simple Einstein model for glasses) would give κ =2 (ref. 56 ), κ<2 implies that fluctuations near jamming are divergently larger than for independent vibrations, in support of their cooperative nature [25] , [56] . Note that if one ignores the fractal phase, an explicit computation erroneously gives κ=1 (ref. 36 ). Also, note that the exponent κ controls the fractal dimension of the basins, as discussed above. The pair correlation function g ( r ) bears a signature of the criticality at the jamming transition. The theory predicts, consistently with the analysis of ref. 57 , that when p →∞, g ( r ) develops an isostatic contact peak characterized by a scaling function ( λ )≡ g ( r )/ g (1) for λ =( r −1) p ( Fig. 4 and Supplementary Note 1 ). It also predicts that the scaling function of the contact peak decays as ( λ )~ λ −2−θ at large λ . The distribution P ( f ) of inter-particle forces in the packing, which is related to the scaling function of the contact peak by (refs 18 , 40 , 57 ), thus also decays as a power law P ( f )~ f θ at small forces. Note that, as observed in ref. 58 , this phenomenon is closely related to what happens to the distribution of frozen fields in the SK model [59] , which is thought to explain the Coulomb gap in interacting electron systems [47] . Beyond the contact peak, the slower decay of pair correlation function follows another power-law g ( r )~( r −1) −α that describes the abundance of quasi-contacts. These scalings of g ( r ) are crucial for determining the mechanical stability of packings [48] , [58] . Perturbing a packing breaks some contacts with small forces, while also forming new contacts from what previously were quasi-contacts. On the basis of this observation, a scaling relation for mechanical stability α =1/(2+ θ ) can be derived [58] . Remarkably, the exponents predicted by our theory, α =0.41269 and θ =0.42311, satisfy this scaling relation to within numerical precision. Previous estimates of these exponents were also obtained by numerical simulation. The quasi-contact exponent α has been measured by several groups in dimension d ranging from 2 to 13, all obtaining roughly α ≈0.4 (refs 39 , 40 , 48 , 57 , 60 ), the most precise estimates being α =0.41(3) (ref. 40 ). The weak force exponent θ is, however, more difficult to measure, and values spanning the interval θ ≈0.2÷0.45 have been reported [40] , [48] . Although the existence of a second exponent θ ′< θ has been shown to affect the tail of P ( f ) (ref. 48 ), its role in determining ( λ ) and its large-dimensional scaling remains to be clarified. Additional numerical simulations are thus needed to test the theory more stringently. 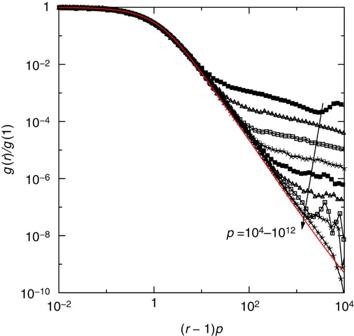Figure 4: Pair correlation function close to jamming. Scaling of the contact peak of the pair correlationg(r). The theory predicts that in the limitp→∞ one hasg(r)/g(1)=(λ) withλ=(r−1)p. Points are numerical data forg(r) ind=4 obtained at several pressuresp=104, 105,…, 1012; the full line is the theoretical prediction. Figure 4: Pair correlation function close to jamming. Scaling of the contact peak of the pair correlation g ( r ). The theory predicts that in the limit p →∞ one has g ( r )/ g (1)= (λ) with λ =( r −1) p . Points are numerical data for g ( r ) in d =4 obtained at several pressures p =10 4 , 10 5 ,…, 10 12 ; the full line is the theoretical prediction. Full size image A prediction for the force distribution P ( f ) at jamming is also available from the theory. However, because this function is not completely determined by the scaling regime, it must be obtained by solving the full equations that describe the marginal phase. Numerically, the function is much easier to measure than P ( f ) because it only depends on structural information, while, in hard spheres, forces must be determined from the collision dynamics. The theoretical prediction for the scaling function (λ) is tested against numerical simulations in Fig. 4 , with very good agreement. We have described the marginal phase that is present below the Gardner transition for hard spheres in d =∞. Using this result we have shown that the jamming transition happens inside the marginal phase and that its low-dimensional criticality is well described by our approach. This analysis opens the way for analytically determining many other properties of jammed packings, such as their shear modulus [61] , and the properties of avalanches [62] . The microscopic explanation of several hitherto mysterious properties of low-temperature glasses might also emerge from this work. (i) A well-attested observation is that glasses that are quenched deeply and rapidly continue to age after the quench, even if the system is well inside the glass phase and there is no activation energy or volume that allows for changes of basin [5] . If the same final pressure is reached with a slower annealing protocol, the subsequent ageing effect is less marked. This observation becomes quite natural if we think in terms of the diagram of Fig. 2 . Metastable states that may be reached with a faster annealing become fractal (that is, undergo a Gardner transition) at pressures much closer to the liquid–glass transition, while the better annealed ones reached with slower protocols only do so at higher pressures. (ii) A related observation is that the existence of a transition from stable to marginal glass along the threshold line (marked by a diamond in Fig. 2 ) might affect the ageing dynamics after a deep and very fast quench [9] , [46] , inducing a change in the ageing properties as a function of the final temperature akin to those observed in some polymer glasses [63] . A more detailed investigation of these effects will require characterizing the off-equilibrium dynamics in the marginal phase [9] , [46] , which at present is only poorly understood. (iii) Another fact that does not fit the standard picture is the observation of dynamical heterogeneities in low-temperature glasses [64] , [65] at timescales much shorter than the inter-basin relaxation. Low-temperature dynamical heterogeneities with a diverging four-point susceptibility are a signature of a fractal phase [30] , while they are expected to be absent within a simple glass basin. Here the theory is well developed, but a detailed comparison with experiments is still missing. (iv) The quantum properties of low-temperature glasses has long been described in terms of a set of tunnelling two-level systems (TLS), characterized by a non-trivial distribution of barriers [66] . The origin of TLS is not understood, but it has been proposed, using schematic models, that TLS might be due to low-energy excitations associated with a marginally stable phase of the kind discussed above [67] . Within our approach, an exact computation of the quantum properties at very low temperatures is viable, and one may hence expect that two-level systems could be put on a first-principle footing. (v) As mentioned in the introduction, Johari-Goldstein processes can be interpreted as transitions between sub-basins belonging to a same metabasin [4] , [5] , [26] . This interpretation naturally explains their many-body origin [68] , but transforming this physical intuition in a theoretically solid explanation requires additional work. Although in the limit d →∞ the equilibrium supercooled liquid region is always far away from the marginal phase, where Johari-Goldstein-like relaxations are expected, we suspect that activated processes, which are absent in d →∞ but play a prominent role in d =3, might bring supercooled liquids much closer to the marginal region. The contribution of Johari-Goldstein processes to glass dynamics may thus be enhanced in d =3 compared with the mean-field prediction. In the d =∞ limit, the barriers controlling inter-basin relaxation should indeed scale as d , and the largest ones, separating sub-basins, as d 1/3 , which suggest the existence of quasi-localized excitations [69] (stringlike, in three dimensions [70] ). Analytical results Results are based on the combination of analytical and numerical methods. Analytical results come from the exact solution of hard spheres in the limit d →∞, which, for convenience, is obtained using the replica method, but any other method would give the same result. The fractal phase is described by a function Δ( y ) for y ∈ [1, y max ], as in the SK model [29] . The cutoff y max ~ p diverges with pressure. With these definitions, Δ EA =Δ( y max ) is the mean square displacement in the smallest sub-basins, where Δ( y ) can be computed by numerically solving a set of coupled integro-differential equations obtained from the replica approach ( Supplementary Note 1 ). Numerical simulations Numerical results are obtained by standard event-driven molecular dynamic simulations in d =3–8 (refs 39 , 40 ). Slow compressions are made using the Lubachevsky-Stillinger algorithm [39] ( Supplementary Note 2 ). How to cite this article: Charbonneau, P. et al. Fractal free energy landscapes in structural glasses. Nat. Commun. 5:3725 doi: 10.1038/ncomms4725 (2014).